Zscan4 restores the developmental potency of embryonic stem cells The developmental potency of mouse embryonic stem (ES) cells, which is the ability to contribute to a whole embryo, is known to deteriorate during long-term cell culture. Previously, we have shown that ES cells oscillate between Zscan4 − and Zscan4 + states, and the transient activation of Zscan4 is required for the maintenance of telomeres and genome stability of ES cells. Here we show that increasing the frequency of Zscan4 activation in mouse ES cells restores and maintains their developmental potency in long-term cell culture. Injection of a single ES cell with such increased potency into a tetraploid blastocyst gives rise to an entire embryo with a higher success rate. These results not only provide a means to rejuvenate ES cells by manipulating Zscan4 expression, but also indicate the active roles of Zscan4 in the long-term maintenance of ES cell potency. Mouse embryonic stem (ES) cells are prototypical pluripotent cells, which are derived from the inner cell mass (ICM) of blastocysts [1] , [2] . The most striking evidence of their pluripotency or high developmental potency (that is, ability to contribute to many tissues in chimeric mice) has been demonstrated by injecting 10–15 ES cells into tetraploid (4N) blastocysts, which produces healthy pups entirely from ES cells [3] . It has been shown that even a single ES cell can form an entire healthy pup, though the success rate was extremely low (0.5%) [4] . Although ES cells have the capacity to maintain their high potency for many cell passages [5] , it is also widely recognized that even ES cells, in long-term culture, gradually lose their potency. It is thus of considerable interest if there is any intervention that can enhance or prolong the high potency of ES cells. Recently, it has been shown that Zscan4 (zinc finger and scan domain-containing protein 4), which is expressed specifically in 2-cell stage embryos [6] and ES cells [6] , [7] , [8] , [9] , is required for the maintenance of genome stability and a normal karyotype in ES cells [7] . Although only a small fraction (1~5%) of undifferentiated ES cells express Zscan4 at a given time [6] , [8] , essentially all of the ES cells in culture undergo the transient Zscan4 + state within nine passages [7] . Undifferentiated ES cells thus oscillate between the Zscan4 − state and the Zscan4 + state, during which dramatic events, including telomere extension, occur [7] . We and others have also shown that Zscan4 can enhance the efficiency and quality of induced pluripotent stem cell (iPSC) formation [10] , [11] . Unlike other iPSC factors, Zscan4 is required only for the initial few days during iPSC formation, suggesting Zscan4’s involvement in epigenetic reprogramming [10] . Given the unusual expression pattern and functions of Zscan4, we hypothesized that more frequent activation of Zscan4 further improves the quality of ES cells, including their developmental potency, in long-term cell culture. Here, we test the notion and demonstrate that ES cells can indeed acquire and maintain higher potency in long-term culture by more frequent activation of Zscan4 than in a normal ES cell condition. We also find that ES cells in the Zscan4 + state show lower potency than ES cells in Zscan4 − state. These data indicate that ES cells can be rejuvenated by going through the transient Zscan4 + state, which lacks the potency temporarily. Zscan4–ERT2 increases the frequency of endogenous Zscan4 + cells Previously, we have shown that constitutive expression of Zscan4 slows down or arrests the proliferation of both ES cells and mouse embryo fibroblast (MEF) cells [10] . We therefore used a plasmid construct pCAG–Zscan4–ERT2, in which a strong ubiquitous promoter CAG [12] drives the expression of an open reading frame (ORF) of Zscan4c fused with a tamoxifen (Tmx)-controlable ERT2 domain [13] ( Fig. 1a ). When we transfected the pCAG–Zscan4–ERT2 plasmid into MC1-ZE3 cells [14] (129S6/SvEvTac strain) carrying an Emerald (green fluorescent protein variant) reporter under the Zscan4 promoter [7] , we were surprised to find that the constitutive expression of Zscan4–ERT2 in ES cells increased the fraction of Em + cells even in the Tmx − condition ( Fig. 1b ). Adding Tmx to the culture media further increased the fraction of Em + cells, but also made the ES cells (both Em + and Em − cells) flatter, resulting in the flattening of ES cell colonies—a deviation from the typical pluripotent ES colony morphology ( Fig. 1b ). The results were further confirmed by quantitative assays for five independent clones: the constitutive expression of Zscan4–ERT2 even in the absence of Tmx caused a threefold increase of Em + cells by flow cytometry analysis ( Fig. 1c ) and a fivefold increase by quantitative reverse transcription PCR (qRT–PCR) analysis ( Fig. 1d ); and the addition of Tmx to the medium caused a further twofold and 1.2-fold increase, respectively ( Fig. 1c ). 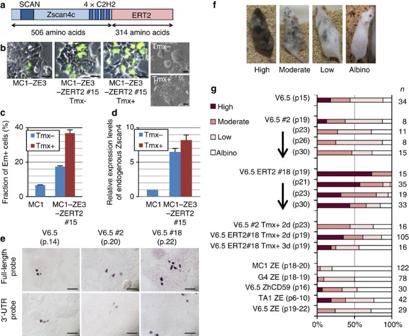Figure 1: Constitutive expression of a Zscan4c–ERT2 fusion protein increases developmental potency. (a) The structure of a Zscan4c–ERT2 fusion protein. Zscan4c contains one SCAN domain and four C2H2 zinc finger domains. (b) Fluorescence microscopy of MC1-ZE3 cells, in which a Zscan4 promoter drives the expression of Emerald marker (left), MC1-ZE3-ZERT2 clone #15 cells, in which the Zscan4c–ERT2 fusion protein is constitutively expressed, cultured in the absence of Tmx (middle), MC1-ZE3-ZERT2 clone #15 cells cultured in the presence of Tmx for 3 days (right). Scale bar, 50 μm. (c) Flow cytometry analysis of MC1–ZE3 ES cells (left, control) and MC1–ZE3–ZERT2 #15 ES cells (right) in the absence or presence of 1 μM Tmx. Em fluorescence levels (average±s.e.m.; n=6) are shown. Note threefold increase of Em+cells by the constitutive expression of a Zscan4c–ERT2 fusion protein even without Tmx. (d) Quantitative RT–PCR analysis of endogenous Zscan4 expression measured by using PCR primer pairs specific for 3′ UTR of Zscan4 in MC1–ZE3 ES cells (left, control) and MC1–ZE3–ZERT2 #15 ES cells (right) in the absence or presence of 1 μM Tmx. The fold induction of endogenous Zscan4 expression levels (average±s.e.m.;n=6) compared with that of control MC1–ZE3 is shown. Note the sixfold increase of endogenous Zscan4 at the RNA level by the constitutive expression of a Zscan4c–ERT2 fusion protein even without Tmx. (e) V6.5 parental ES cells (passage number 14), V6.5 ZERT2 #2 (p.20), V6.5 ZERT2 #18 (p.22) ES cell colonies after whole-mount RNAin situhybridization of a Zscan4 full-length probe (which detects both endogenous and exogenous Zscan4 RNAs: upper panel) or a Zscan4 3’-UTR probe, which detects only endogenous Zscan4 RNAs. Scale bar, 100 μm. (f) Representative coat colours of chimeric mice generated by injecting various ES cells into blastocysts. Higher chimerism represents higher contribution of injected ES cells to mice, indicating higher developmental potency of the ES cells. (g) Percentage distribution of chimerism levels among ‘n’ number of mice born from various ES cell lines. Figure 1: Constitutive expression of a Zscan4c–ERT2 fusion protein increases developmental potency. ( a ) The structure of a Zscan4c–ERT2 fusion protein. Zscan4c contains one SCAN domain and four C2H2 zinc finger domains. ( b ) Fluorescence microscopy of MC1-ZE3 cells, in which a Zscan4 promoter drives the expression of Emerald marker (left), MC1-ZE3-ZERT2 clone #15 cells, in which the Zscan4c–ERT2 fusion protein is constitutively expressed, cultured in the absence of Tmx (middle), MC1-ZE3-ZERT2 clone #15 cells cultured in the presence of Tmx for 3 days (right). Scale bar, 50 μm. ( c ) Flow cytometry analysis of MC1–ZE3 ES cells (left, control) and MC1–ZE3–ZERT2 #15 ES cells (right) in the absence or presence of 1 μM Tmx. Em fluorescence levels (average±s.e.m. ; n=6) are shown. Note threefold increase of Em + cells by the constitutive expression of a Zscan4c–ERT2 fusion protein even without Tmx. ( d ) Quantitative RT–PCR analysis of endogenous Zscan4 expression measured by using PCR primer pairs specific for 3′ UTR of Zscan4 in MC1–ZE3 ES cells (left, control) and MC1–ZE3–ZERT2 #15 ES cells (right) in the absence or presence of 1 μM Tmx. The fold induction of endogenous Zscan4 expression levels (average±s.e.m. ; n =6) compared with that of control MC1–ZE3 is shown. Note the sixfold increase of endogenous Zscan4 at the RNA level by the constitutive expression of a Zscan4c–ERT2 fusion protein even without Tmx. ( e ) V6.5 parental ES cells (passage number 14), V6.5 ZERT2 #2 (p.20), V6.5 ZERT2 #18 (p.22) ES cell colonies after whole-mount RNA in situ hybridization of a Zscan4 full-length probe (which detects both endogenous and exogenous Zscan4 RNAs: upper panel) or a Zscan4 3’-UTR probe, which detects only endogenous Zscan4 RNAs. Scale bar, 100 μm. ( f ) Representative coat colours of chimeric mice generated by injecting various ES cells into blastocysts. Higher chimerism represents higher contribution of injected ES cells to mice, indicating higher developmental potency of the ES cells. ( g ) Percentage distribution of chimerism levels among ‘ n ’ number of mice born from various ES cell lines. Full size image To further investigate this unexpected result, we transfected the pCAG–Zscan4–ERT2 plasmid into V6.5 ES cells derived from an F1 hybrid strain (C57BL/6 × 129/Sv), which has been extensively used for testing developmental potency [4] , [15] , and isolated multiple cell clones named V6.5 ZERT2 (ref. 10) [10] . Based on qRT–PCR analysis of Zscan4 ORF, we selected clone #18 for the highest Zscan4 expression levels, clones #7 and #10 for the second and third highest Zscan4 levels, and clone #2 with a background Zscan4 level [10] . Based on genotyping by PCR, clone #2 did not have any copies of the pCAG–Zscan4–ERT2 plasmid, and was thus used as a control (V6.5 #2). To check if the frequency of Zscan4 + cells is increased even in the Tmx − condition, we carried out whole-mount in situ hybridization using a full-length Zscan4c probe to detect both endogenous and exogenous copies of Zscan4 as well as a 3′-UTR Zscan4c probe to detect only endogenous Zscan4. The results showed an ~3-fold increase of the number of Zscan4 + cells in V6.5 ZERT2 ES cell clones (#10 and #18) in the absence of Tmx compared with the usual level of Zscan4 + cells in the control cells (V6.5 and V6.5 #2) ( Fig. 1e , Supplementary Fig. S1 ). Similarly, the number of V6.5 ZERT2#18 cells expressing the Zscan4 protein was ~3-fold greater than the control V6.5 cells ( Supplementary Fig. S2a–c ). The Zscan4 protein detected here by antibodies against Zscan4 was most likely endogenous Zscan4 proteins, because they constituted only ~3% of cells expressing the Zscan4–ERT2 fusion protein detected by antibodies against the ERT2 domain ( Supplementary Fig. S2d ). The effect of Zscan4–ERT2 without its usual ligand Tmx may be partially explained by the presence of ~25% of Zscan4–ERT2 proteins leaked in nucleus in the absence of Tmx, although more Zscan4–ERT2 proteins (~56%) were translocated from cytoplasm to nucleus in the presence of Tmx, as expected ( Supplementary Fig. S3 ). Taken together, the use of constitutively expressing the Zscan4–ERT2 fusion protein without Tmx became an unexpected, but attractive, strategy to enhance the naturally occurring Zscan4 effects by increasing the frequency of endogenous Zscan4 activation, resulting in more Zscan4 + cells in culture. Zscan4–ERT2 enhances developmental potency of ES cells To assess the effects of Zscan4–ERT2 on the developmental potency of ES cells, we injected various ES cells into mouse blastocysts, transferred them to uteri and followed their development. The extent of ES cell potency was assessed by percentage chimerism in the pups based on coat colours: high (>70% chimerism), moderate (40–70%), low (<40%) and albino (0%) ( Fig. 1f ). A V6.5 parental ES cell line at its early passage (passage 15; p15) showed 18% high, 29% moderate and 41% low chimerism, which are within the standard range for F1 hybrid ES cell lines ( Fig. 1g ). It is known that the developmental potency of ES cells generally becomes lower after multiple passages and/or plasmid transfection/drug selection. As expected, compared with a V6.5 parental ES cell line, the control V6.5 #2 ES cell line, which did not carry Zscan4–ERT2 but was generated after transfection and drug selection, showed a slightly lower overall potency, which was further reduced over multiple passages (p23, p26 and p30) ( Fig. 1g ). By contrast, V6.5 ZERT2 #18 ES cells showed much higher developmental potency than parental V6.5 and control V6.5 #2 ES cells: 73% high and 27% moderate chimerism at passage 19 ( Fig. 1g ). Even more surprising was that such a high level of potency was maintained for an extended period of time and passages: for example, even at passage 30, more than 40% of pups derived from V6.5 ZERT2 #18 ES cells showed high chimerism, whereas none of the pups derived from control V6.5 #2 ES cells showed high chimerism ( Fig. 1g ). We tested five other ES cell lines of different genetic backgrounds and found that potency-wise, none of these ES cell lines could even come close to V6.5 ZERT2 #18 lines ( Fig. 1g ). Consistent with the flatter ES cell morphology mentioned above, the exposure to Tmx for 2 to 3 days lowered the potency of both V6.5 #2 and V6.5 ZERT2 #18 ES cells relative to that in the Tmx − condition ( Fig. 1g ). The developmental potential of these ES cells were also assessed by the efficiency of germline transmission from the chimeric mice ( Supplementary Table S1 ). Consistent with the developmental potency assessed by the chimerism, the V6.5 ZERT2#18 cell clone showed the highest overall efficiency for the germline transmission (22%) compared with other cell clones including the control V6.5 ES cells (7%). Testing developmental potency by 4N complementation It is widely recognized that the ultimate test for developmental potency is to see if ES cells alone injected into tetraploid (4N) blastocysts become an entire mouse [16] . We thus tested the potency of ES cells by injecting 10 to 15 cells into 4N blastocysts. Compared with early-passage V6.5 ES cells reported previously, which have achieved 15–25% pups alive at term [15] , V6.5 ES cells at passage 18–19 only produced 3% live embryos ( Table 1 ). By contrast, V6.5 ZERT2 #18 ES cells showed a much higher success rate—43% live embryos even at passage 19 ( Table 1 ). Similarly, one of two other independent clones tested also showed a high success rate of producing live embryos ( Table 1 : V6.5 ZERT2#10). Interestingly, one common feature of these two clones was an upregulation of endogenous Zscan4 expression ( Supplementary Fig. S1a ). Table 1 Tetraploid (4N) complementation assays confirm the higher potency of ES cells expressing a Zscan4c–ERT2 fusion protein. Full size table To compare the high success rate of V6.5 ZERT2 #18 cells with those of the best ES cells possible, we freshly isolated ES cells from blastocysts with the same genetic background—F1 hybrid of C57BL/6J × 129S6/SvEvTac, and cultured them in the best conditions currently available [17] ( Supplementary Tables S2 and S3 , Fig. S4 ). Of the 13 ES lines established, one ES line, named ‘TA1’, showed the highest efficiency (60%) in producing live embryos, although its potency quickly decreased over multiple passages ( Table 1 ). Overall, these results indicate that the developmental potency of V6.5 ZERT2 #18 ES cells even at a higher passage number was comparable to that of freshly isolated early-passage ES cells. To exclude the possibility that Zscan4–ERT2 affects only F1 hybrid ES cell lines, we generated MC2 ZERT2 ES cells by transfecting a pCAG–Zscan4–ERT2 plasmid into an MC2 ES cell line (C57BL/6J) [14] . Consistent with the reported low potency of C57BL/6J-derived ES cells [15] , [18] , both MC2 ES cells at passage 17 and genetically modified MC2 ES cells at passage 12–13 did not produce any live embryos ( Table 1 ). By contrast, several independent MC2 ZERT2 cell lines successfully achieved the production of 4–15% live embryos, respectively, even after 17 passages ( Table 1 ). The unusually high developmental potency of V6.5 ZERT2 #18 cells prompted us to further examine the potency of single ES cells by the 4N complementation assay. It has been shown once that even a single ES cell can form a live pup, although the success rate is extremely low (1 mouse/192 injected blastocysts: 0.5%) [4] . 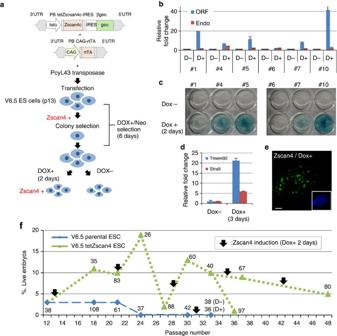Figure 2: Forced expression of Zscan4 enhances developmental potency of ES cells. (a) Schematic presentation of experimental procedure. (b) Expression levels of Zscan4 (endogenous and ORF) in Dox+and Dox−conditions in G418-selected clones. Error bars indicate s.e.m.,n=3. (c) Forced expression of βgeo in Dox+and Dox−conditions. (d) Induction of Stra8 and Tmem92 (Zscan4-downstream genes) in Dox+condition. Error bars indicate s.e.m.,n=3. (e) Forced expression of Zscan4 protein detected by immunohistochemistry. Scale bar, 100 μm. (f) Assessment of developmental potency of ES cells by 4N complementation assays. The number shown near each data point indicates the number of transferred blastocysts. D+and D−at p33 indicate the results for cells treated with Dox+and Dox−at p31, respectively. As expected from the fact that we used the same cell line as the one used for the earlier study [4] , out of 71 single V6.5 ES cells (p18) injected, only 1 live embryo (1%) was obtained ( Table 2 ). Similarly, of 77 single control V6.5 #2 ES cells, none of them produced live embryos ( Table 2 ). By contrast, of the 44 tetraploid blastocysts that received a single V6.5 ZERT2 #18 cell, 3 (7%) became complete embryos, 2 (5%) of which were alive at the time of dissection ( Table 2 ). This unusually high level of potency for V6.5 ZERT2 #18 ES cells was indeed comparable to that of early-passage TA1 ES cells with 4% live embryos ( Table 2 ). Overall, these results indicate that the pCAG–Zscan4–ERT2 construct can be used as a tool to enhance the developmental potency of ES cells. Table 2 Tetraploid (4N) complementation assays confirm the higher potency of ES cells expressing a Zscan4c–ERT2 fusion protein. Full size table Forced expression of Zscan4 enhances developmental potency Results obtained using Zscan4–ERT2 fusion protein thus far indicate that increasing the frequency of Zscan4 + cells can restore and maintain the developmental potency of ES cells. To test whether the Zscan4 gene itself can cause this effect, we established V6.5 ES cell lines carrying a doxycycline (Dox)-inducible Zscan4c ORF linked to IRES-βgeo ( Fig. 2a ). After confirming the high Dox inducibility of exogenous Zscan4 by qRT–PCR ( Fig. 2b ) and βgeo by LacZ staining ( Fig. 2c ), we selected V6.5 tetZscan4 #10 (clone #10) for further studies. The qRT–PCR ( Fig. 2b ) and Emerald-reporter ( Supplementary Fig. S5 ) assays showed that the Dox-induced exogenous Zscan4 expression also increased the number of endogenous Zscan4 + cells by ~3-fold. Dox-dependent upregulation of two Zscan4-inducible genes— Tmem92 and Stra8 —was also confirmed ( Fig. 2d ). Although the antibodies against Zscan4 cannot distinguish between endogenous and exogenous Zscan4 proteins in this case, immunohistochemical analyses confirmed that 2-day Dox treatment increased the number of cells expressing Zscan4 proteins (~50% of cells), which subsequently declined to the basal level by 1 day after Dox withdrawal ( Fig. 2e ; Supplementary Fig. S6 ). These results indicate that 2-day Dox treatment causes transient expression of Zscan4 in ~50% of V6.5 tetZscan4 #10 cells. Figure 2: Forced expression of Zscan4 enhances developmental potency of ES cells. ( a ) Schematic presentation of experimental procedure. ( b ) Expression levels of Zscan4 (endogenous and ORF) in Dox + and Dox − conditions in G418-selected clones. Error bars indicate s.e.m., n =3. ( c ) Forced expression of βgeo in Dox + and Dox − conditions. ( d ) Induction of Stra8 and Tmem92 (Zscan4-downstream genes) in Dox + condition. Error bars indicate s.e.m., n =3. ( e ) Forced expression of Zscan4 protein detected by immunohistochemistry. Scale bar, 100 μm. ( f ) Assessment of developmental potency of ES cells by 4N complementation assays. The number shown near each data point indicates the number of transferred blastocysts. D + and D − at p33 indicate the results for cells treated with Dox + and Dox − at p31, respectively. Full size image Developmental potency was assayed by injecting 10–15 ES cells into individual 4N blastocysts and by examining the presence of live embryos at E13.5 (see above). Parental V6.5 ES cells (p12) as a control showed its standard potency (that is, ~3% live embryos), which deteriorated to 0% by passage 24 and continued to be 0% at passage 30 ( Fig. 2f ). As expected, Dox treatment for 2 days at passage 31 did not change the potency of V6.5 ES cells ( Fig. 2f ). By contrast, the initial exposure to Zscan4 by 6-day Dox/G418 treatment for clone isolation increased the potency from 3% (p12) to 11% (p18). By passage 21, the potency was slightly decreased, but another exposure to Zscan4 by 2 days of Dox treatment increased the potency further to 19% (p24). Subsequently, the potency declined again to 2% (p27), but yet another exposure to Zscan4 by 2-day Dox treatment increased the potency to 13% (p30). Similar trends continued for two more cycles of forced Zscan4 expression that we tested. Even at passage 48, the potency was 5%, which was more than passages 12–21 of the control V6.5 ES cells ( Fig. 2f ). As expected, we found that Dox-inducible Nanog [19] did not increase the developmental potency of ES cells, suggesting that this is indeed a unique function of Zscan4 ( Supplementary Fig. S7 ). Taken together, these results demonstrate that the forced and transient expression of Zscan4 itself could enhance and maintain the developmental potency of ES cells in long-term culture. Zscan4 + ES cells do not show higher developmental potency Expression of Zscan4 in the 2-cell embryos, but not in the ICM, suggests that ES cells are a mixed population of ~5% of 2-cell-like cells (that is, Zscan4 + state) and ~95% of ICM-like cells (that is, Zscan4 − state) [6] . As it has been shown that by nuclear transplantation (cloning) the 2-cell nucleus has a higher developmental potential than the ICM nucleus [20] , [21] , it is tempting to speculate that the Zscan4 + state represents high-potential stem cells among the regular ES cell population. It is also conceivable that the enhancement of potency in ES cells after increasing the frequency of Zscan4 activation or after exposing ES cells to Zscan4 protein might simply be owing to the increased presence of Zscan4 + cells in the culture. To test this notion, we first sorted G4ZE#17 cells into Em + and Em − cells by fluorescence-activated cell sorting and tested their developmental potency ( Supplementary Table S4 ). Compared with non-sorted cells (62% chimerism), both Em − cells (2% chimerism) and Em + cells (0% chimerism) showed very low chimerism. To test another cell clone and avoid possible cell damage caused by cell sorting, we separated the MC1ZE cells manually by mouth pipetting in the order of Em + (under ultraviolet light), Em − (under ultraviolet light) and Em + /Em − mixed population (without ultraviolet light). To collect sufficient number of cells for blastocyst injections of 10–15 ES cells, Em + cells included not only the highest Em + expression but also the medium–low Em + expression. 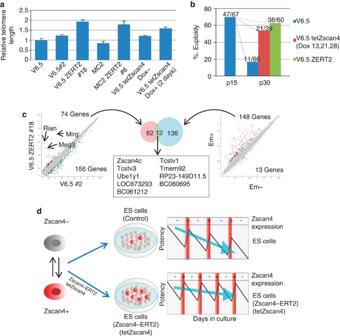Figure 3: Molecular features of ES cells expressing Zscan4–ERT2 and a proposed mode of Zscan4 actions. (a) Constitutive presence of Zscan4–ERT2 and forced expression of Zscan4 made telomeres longer than controls in both F1-hybrid (129/C57BL/6)-derived ES cells (V6.5) and C57BL/6-derived ES cells (MC2). Telomere lengths (average±s.e.m.;n=3) are shown. (b) Constitutive presence of Zscan4–ERT2 and forced expression of Zscan4 maintained better karyotype in long-term culture of ES cells. (c) Comparisons of global expression profiles between V6.5 ZERT2 #18 ES cells and V6.5 #2 control ES cells (left scatter plot) and between MC1 Em+(Zscan4+) ES cells and Em−(Zscan4−) ES cells (right scatter plot). Red and green dots represent genes that show expression differences with statistical significance (false discovery rate <0.05 and fold change >2). Venn diagram showing the overlap between genes that are more highly expressed in V6.5 ZERT2 #18 cells than V6.5 #2 cells, and genes that are more highly expressed in Em+(Zscan4+) cells than Em−(Zscan4−) cells (centre). (d) A proposed model. Upper panel: ES cells oscillate between Zscan4−and Zscan4+states, resulting in the normal ES cells with only 1–5% of Zscan4+cells. While in Zscan4−state, the potency of ES cells gradually decreases, which is restored to some extent by transient activation of Zscan4 (Zscan4+state). However, the potency of ES cells still decreases during the long-term culture. Lower Panel: when the Zscan4 is more frequently activated by expressing an exogenous Zscan4, ES cells are rejuvenated more frequently, resulting in the longer maintenance of the high developmental potency. Based on the coat colours, we found that Em − ES cells were able to contribute to the tissues of chimeric mice at higher rate (75%) than Em + ES cells (31%) ( Table 3 ). Owing to the order of cell picking, Em + /Em − mixed cells and Em − cells were exposed to the ultraviolet light longer than Em + cells; therefore, it is unlikely that the reduced potency of Em + cells was caused by the ultraviolet-induced cell damage. To test yet another cell clone, we generated and assessed the developmental potency of V6.5 ZE cells (clone #17) by transfecting a pZscan4–Emerald vector [7] into V6.5 ES cells. We separated V6.5 ZE cells into Em + or Em − cells manually by mouth pipetting, injected single ES cells into 2N blastocysts and observed the subsequent embryo development. Based on the coat colours, we found that Em − ES cells were able to contribute to the tissues of chimeric mice at a relatively high rate (31%), whereas Em + ES cells were not ( Table 3 ). The results indicate that, contrary to our expectations, Zscan4 + cells are not associated with high developmental potency compared with Zscan4 − cells. Consistent with this notion, we observed in at least one instance that too frequent activation of Zscan4, resulting in more Zscan4 + cells in culture, lowered the average potency of ES cells ( Supplementary Fig. S8 : TA1–ZERT2). Taken together, these data suggest that the Zscan4 + state is the process that restores potency, but the process itself (that is, Zscan4 + state) has no or low potency. Table 3 Zscan4 + cells do not show higher developmental potency. Full size table Characterization of ES cells with potency enhanced by Zscan4 In our earlier work, we have shown that Zscan4 extends telomeres and is responsible for the maintenance of normal karyotype of ES cells [7] . We therefore examined if the restoration of developmental potency of ES cells by transient activation of Zscan4 can be simply explained by better karyotype and longer telomeres. We indeed found that the lengths of telomeres were twofold longer in V6.5 ZERT2 #18 (p30) compared with control V6.5 #2 ( Fig. 3a ). This held true also for MC2 ES cells: MC2 ZERT2 #6 (p23) showed >2-fold longer than control MC2 ES cells ( Fig. 3a ). Figure 3: Molecular features of ES cells expressing Zscan4–ERT2 and a proposed mode of Zscan4 actions. ( a ) Constitutive presence of Zscan4–ERT2 and forced expression of Zscan4 made telomeres longer than controls in both F1-hybrid (129/C57BL/6)-derived ES cells (V6.5) and C57BL/6-derived ES cells (MC2). Telomere lengths (average±s.e.m. ; n =3) are shown. ( b ) Constitutive presence of Zscan4–ERT2 and forced expression of Zscan4 maintained better karyotype in long-term culture of ES cells. ( c ) Comparisons of global expression profiles between V6.5 ZERT2 #18 ES cells and V6.5 #2 control ES cells (left scatter plot) and between MC1 Em + (Zscan4 + ) ES cells and Em − (Zscan4 − ) ES cells (right scatter plot). Red and green dots represent genes that show expression differences with statistical significance (false discovery rate <0.05 and fold change >2). Venn diagram showing the overlap between genes that are more highly expressed in V6.5 ZERT2 #18 cells than V6.5 #2 cells, and genes that are more highly expressed in Em + (Zscan4 + ) cells than Em − (Zscan4 − ) cells (centre). ( d ) A proposed model. Upper panel: ES cells oscillate between Zscan4 − and Zscan4 + states, resulting in the normal ES cells with only 1–5% of Zscan4 + cells. While in Zscan4 − state, the potency of ES cells gradually decreases, which is restored to some extent by transient activation of Zscan4 (Zscan4 + state). However, the potency of ES cells still decreases during the long-term culture. Lower Panel: when the Zscan4 is more frequently activated by expressing an exogenous Zscan4, ES cells are rejuvenated more frequently, resulting in the longer maintenance of the high developmental potency. Full size image The standard low-resolution karyotype analysis showed that the karyotypes of V6.5 ZERT2#18 (p30) and V6.5 tetZscan4#10 (p30; Dox treated for 2 days at p13, p21 and p28) were better than control V6.5#2 (p30) ( Fig. 3b ). With the high-resolution G-banding karyotype analysis, the control V6.5#2 (p30) exhibited 72% tetraploid and 28% interstitial deletions and isochromosome 8, resulting in 0% normal karyotype (0 normal karyotype out of 58 spreads analysed), whereas V6.5 ZERT2#18 (p30) showed 100% normal karyotype (18 normal karyotypes out of 18 spreads analysed) ( Supplementary Fig. S9 , Table S5 ). The high-resolution G-banding analysis also revealed that V6.5 tetZscan4#10 (p30; Dox treated for 2 days at p13, p21 and p28) exhibited 0% tetraploid and 89% isochromosome 8, resulting in only 11% normal karyotype (2 normal karyotypes out of 18 spreads analysed); however, additional 2-day Dox treatment before the G-banding analysis improved the karyotype, resulting in 63% normal karyotype (12 normal karyotypes out of 19 spreads analysed) ( Supplementary Fig. S9 , Table S5 ). Taken together, telomere extension and karyotype maintenance account for at least a part of the enhanced potency caused by Zscan4. To further understand the molecular mechanisms of Zscan4-mediated restoration of developmental potency, we compared the global gene expression profiles of these cells ( Fig. 3c ; Supplementary Tables S6–S8 ). Zscan4 and other key Zscan4-related genes, such as Tcstv1/3 (Struwe, M. and Solter, D., GenBank/EMBL/DDBJ accession AF067057.1.) [22] , Eif1a , Tho4 , Arginase II , GM428 , AF067063 , EG668777 , RP23-149D11.5 , BC061212 and EG627488 , were more highly expressed in Zscan4 + cells than in Zscan4 − cells ( Fig. 3c ; Supplementary Table S6 ). We also found that these genes are indeed expressed in Zscan4 + ES cells ( Supplementary Fig. S10 ) and are expressed specifically in early preimplantation embryos ( Supplementary Fig. S11 ). Consistent with the more frequent presence of Zscan4 + cells in V6.5 ZERT2 #18 ES cells, these genes were slightly upregulated in V6.5 ZERT2 #18 ES cells in the Tmx − condition ( Fig. 3c , Supplementary Table S7 ). However, more dramatic upregulation was observed for genes in the well-known imprinted cluster: Rian (192-fold), Mirg (92-fold) and Meg3 (45-fold). Previously, these genes were implicated as markers for ES cells with higher developmental potency [23] , [24] . These results suggest that transient activation of Zscan4 made dramatic epigenetic changes to the ES cell genome, which persisted for a long time even without Zscan4 expression. However, it remains to be clarified whether these imprinted genes have a role in the function of Zscan4, as their strong upregulation were not observed in Zscan4 + ES cells and V6.5 tetZscan4 ES cells. Given the beneficial effects of Zscan4 on ES cells, it is of particular interest to find if any of the cell culture conditions that are known to enhance the pluripotency of ES cells can replace exogenous Zscan4. As a first step to address this issue, we tested the knockout serum replacement (KSR)-supplemented medium, which is widely used for the efficient derivation and maintenance of ES cells [25] , and the defined medium supplemented with the two inhibitors (2i) of the mitogen-activated protein kinase (ERK1/2) cascade and of glycogen synthase kinase 3, which is known to provide an optimal culture environment for mouse ES cells [26] . We found that the responses to the KSR or 2i condition were slightly different between V6.5 (C57BL/6 × 129/Sv) and MC1 (129S6/SvEvTac) ES cells ( Supplementary Fig. S12 ). In V6.5 ES cells, the 2i condition did not increase the number of Em + cells in 2 days, but increased by ~3-fold in 5 days; in MC1 ES cells, the 2i condition increased the number of Em + cells by ~2-fold in 2 days, but reduced to the original level in 5 days. The KSR medium showed similar trends with slightly stronger responses than the 2i condition. The combination of the KSR and 2i conditions showed only a modest additional increase. We also found that the KSR medium indeed increased the expression levels of Zscan4-related genes by day 5, but the 2i condition did not change the expression levels of these genes. Interestingly, the expression of so-called pluripotency genes ( Rian and Gtl2 ) was not induced by neither the KSR nor 2i condition, whereas these genes were highly induced in V6.5ZERT2#18 cells based on our microarray data ( Supplementary Table S7 ). Based on these results, the KSR medium seems to be a possible candidate to replace the exogenous Zscan4; however, relatively fast decline of the developmental potency of the aforementioned TA1 ES cells, which were indeed derived and maintained in the KSR medium all the time ( Table 1 ; Supplementary Fig. S8 ), indicates that the exogenous Zscan4 cannot be substituted by simply the KSR medium. It is known that ES cells oscillate between Zscan4 − and Zscan4 + states [7] , leading to the presence of 1–5% Zscan4 + cells in an ES cell culture at a given time [6] , [7] , [8] . Here, we have shown that the constitutive presence of Zscan4–ERT2, without its usual activator Tmx, can increase the frequency of ES cells in the Zscan4 + state, resulting in an increase of the developmental potency of ES cells. We have also shown that similar effects can be obtained by the periodic and transient overexpression of Zscan4 in a Dox-inducible system. The enhanced potency of ES cells by more frequent activation of Zscan4 than usual indicates that the interval of transient Zscan4 activation in the standard ES cell culture may be longer than the optimal interval ( Fig. 3d ). This suggests that ES cells steadily lose their developmental potency, which can be rapidly restored by the transient activation of Zscan4, although the frequency is less than optimal ( Fig. 3d ). ES cells cultured in the accelerated Zscan4 activation cycle show improved chimerism and potency, which are demonstrated by high contribution to chimeric mice and efficient production of a whole mouse from a single ES cell. These ES cells also show longer telomeres, better karyotypes and upregulation of imprinted genes previously implicated for higher developmental potency of ES cells. Overall, the introduction of Zscan4–ERT2 provides an effective means to maintain or increase (rejuvenate) the developmental potency of pluripotent stem cells in long-term cell culture. Interestingly, our results show that the enhanced potency of ES cells with more frequent Zscan4 activation is not merely owing to the presence of more Zscan4 + cells in culture: Zscan4 + cells showed no or lower potency than Zscan4 − cells in the standard potency assay, that is, injecting into blastocysts. The results indicate that the potency of ES cells can be enhanced when ES cells experience a transient Zscan4 + state, which is in the middle of undergoing dramatic changes in their epigenetic status, and thus is not potent. This seems to be consistent with our earlier findings: (i) drastic changes, including rapid telomere extension by telomere sister chromatid exchange [7] , are occurring in ES cells in the Zscan4 + state; (ii) forced and constitutive expression of Zscan4 in ES cells and MEF cells slows down or arrests their proliferation [10] ; (iii) the forced expression of Zscan4 for the initial few days enhances the efficiency of iPSC formation [10] . Recently, it has been reported that a rare population of ES cells that express endogenous retroviruses and 2-cell embryo genes possesses expanded fate potential with the ability to contribute to both embryonic and extraembryoic tissues [27] . It appears that these rare cells are essentially the same as Zscan4 + cells, which also express Tcstv1/3 and other preimplantation genes highly and show a similar oscillatory appearance [7] . However, it remains to be clarified why two seemingly identical rare cell populations differ in their developmental potency. ES cell culture MC1 ES cells [14] derived from 129S6/SvEvTac and MC2 ES cells [14] derived from C57BL/6J were purchased from the Transgenic Core Laboratory of Johns Hopkins University School of Medicine, Baltimore, MD, USA. V6.5 ES cells [15] derived from an F1 hybrid strain (C57BL/6 × 129/Sv) were purchased from Thermo Scientific Open Biosystem. All ES cell lines, except for TA1 ES cell line (see below), were cultured at 37 °C in 5% CO 2 in the complete ES medium as previously described [7] : DMEM (Gibco), 15% fetal bovine serum (FBS) (Atlanta Biologicals), 1,000 U ml −1 leukaemia inhibitory factor (ESGRO, Chemicon), 1 mM sodium pyruvate, 0.1 mM non-essential amino acids, 2 mM GlutaMAX, 0.1 mM beta-mercaptoethanol and penicillin/streptomycin (50 U/50 μg ml −1 ). For all cell lines, medium was changed daily and cells were passaged every 2 to 3 days routinely. Derivation of TA1 ES cell line C57BL/6J females (The Jackson Laboratory) and 129S6/SvEvTac males (Taconic) were naturally mated to collect 2-cell embryos, which were then cultured in the KSOM medium for 3 days at 37 °C in 5% CO 2 . Resulting blastocysts were transferred onto MEF feeder cells treated with Mitomycin C (Sigma) and cultured for 7 days in the complete ES medium after replacing 15% FBS with 15% KSR (Invitrogen) and adding 50 nM PD98059 (MEK1 inhibitor). After picking ICM clumps and dissociating them by Accutase (Millipore), they were seeded onto fresh feeder cells and cultured in the same conditions for additional 7 days. Subsequently, TA1 ES cells were cultured in the same KSR-containing medium without MEK1 inhibitor. Newly derived ES cell lines were directly tested for their developmental potency by 4N complementation (see below). pCAG–Zscan4–ERT2 vector construction Genes collectively called Zscan4 consist of six paralogous genes and three pseudogenes clustered on a ~850 kb region of chromosome 7 (ref. 6) [6] . Among six paralogs named Zscan4a to Zscan4f, the ORFs of Zscan4c, Zscan4d and Zscan4f are very similar to each other and encode a SCAN domain and four zinc finger domains [6] . To construct a pCAG–Zscan4–ERT2 plasmid, an entire ORF (506 amino acids) of mouse Zscan4c gene [6] was fused with ERT2 (ref. 13) [13] (314 amino acids) and cloned into XhoI/NotI sites of pPyCAG-BstXI-IP (a gift from Dr Hitoshi Niwa). The resultant plasmid vector expresses Zscan4c–ERT2 fusion protein–IRES–Puromycin-resistant protein under a strong CAG promoter [12] . Generation of ZE (Emerald reporter) and ZERT2 ES cell clones ES cells were grown in 6-well plates. For ZE ES cell clones, 5 × 10 5 ES cells in suspension were transfected with 1 μg of a linearized pZscan4–Emerald vector [7] using Effectene (Qiagen) according to manufacturer’s protocol, into various cell lines—MC1, G4 (129S6/SvEvTac × C57BL/6Ncr), TA1 and V6.5, and plated in 100 mm dishes. After selecting with 5 μg ml −1 blasticidin for 8 days, resulting ES cell colonies were picked, expanded and frozen for further analysis. For ZERT2 ES cell clones, 5 × 10 5 ES cells in suspension were cotransfected with 0.5 μg of a linearized pCAG–Zscan4–ERT2 vector and 0.5 μg of PL452 (PGK promoter-Neo) [28] using Effectene, and plated in 100 mm dishes. After selecting with G418 for 8 days, resulting ES cell colonies were picked, expanded and frozen for further analysis. Generation of tet-Zscan4c ES cell clones A PB–TET–Zscan4c–IRES–βgeo vector was constructed as previously described [10] . In brief, an ORF of Zscan4c was PCR-amplified from a pCAG–Zscan4–ERT2 vector by using a high-fidelity DNA polymerase (Pfx50 or Platinum Pfx from Invitrogen) and attB1/2 primers and cloned into a pDONR221 vector (Invitrogen). Subsequently, the DNA fragment was inserted into a PB–TET–IRES–βgeo destination vector thorough the Gateway System (Invitrogen). Using Effecten, V6.5 ES cells were transfected with 0.7 μg of each plasmid: pCyL43 [29] (Sanger Institute), PB-CAG-rtTA and PB-TET-Zscan4c. After 24 h, cells were fed with the complete ES medium with Dox (1.5 μg ml −1 ) and G418 (400 μg ml −1 ) for 6 days. Colonies were picked after 7 days post Dox induction and propagated as tet-Zscan4c ES cells in the complete ES medium. Quantitative reverse transcription PCR RNA was isolated from cells by TRIzol (Invitrogen) in biological triplicate. One microgram of total RNA was reverse transcribed by SuperScript III (Invitrogen) following the manufacturer’s protocol. Hundred nanogram of oligo dT primers (Promega) was used per reaction. For qPCR, SYBR green master mix (Applied Biosystems) was used following the manufacturer’s protocol. Ninety-six-well optical plates with a 25 μl total reaction volume were used, 10 ng of complementary DNA was used per well. Plates were run on 7300 or 7500 system (Applied Biosystems). Fold induction was calculated by the ΔΔCt method [30] using H2A as normalizer. A list of qPCR primer sequences can be found in Supplementary Table S9 . RNA isolation and qPCR analysis in preimplantation embryos Four to 6-week-old B6D2F1 female mice were superovulated with 5 IU of PMSG (Sigma) and 5 IU of hCG (Sigma). Eggs or embryos for qRT–PCR experiments were collected after 20, 23, 30, 43, 55, 66, 80 and 102 h post hCG injection for MII, 1-cell, early and late 2-cell, 4-cell, 8-cell, morula and blastocyst embryos, respectively. Three sets of ten synchronized eggs or embryos were stored in liquid nitrogen and mechanically ruptured by a freeze/thaw step for the cDNA preparation template. Oligo-dT primers and SuperScript III Reverse Transcriptase (Invitrogen) were used according to the manufacturer’s instruction. Analysis was performed on the ABI 7300 Fast Real Time PCR system (Applied Biosystems). A list of qPCR primer sequences can be found in Supplementary Table S9 . Data were normalized by Chuk [31] with the ΔΔCt method [30] . RNA in situ hybridization Whole-mount in situ hybridization was done as previously described [8] . Briefly, ES cells in triplicates, grown for 3 days, were fixed in 4% paraformaldehyde at 4 °C overnight. After digestion with proteinase K, cells were hybridized with 1 μg ml −1 digoxigenin-labelled riboprobe at 62 °C overnight. Cells were then washed, blocked, incubated with alkaline phosphatase-conjugated anti-digoxigenin antibody and incubated with NBT/BCIP detection buffer for 30 min or overnight. Microarray analysis DNA microarray analyses were carried out as described [32] . Briefly, universal Mouse Reference RNA (Stratagene) were labelled with Cy5-dye, mixed with Cy3-labeld samples and used for hybridization on the NIA Mouse 44K Microarray v2.2 (ref. 33) [33] (manufactured by Agilent Technologies #014117). The intensity of each gene feature was extracted from scanned microarray images using Feature Extraction 9.5.1.1 software (Agilent Technologies). Microarray data analyses were carried out by using an application developed in-house to perform analysis of variance and other analyses (NIA Array Analysis software; http://lgsun.grc.nia.nih.gov/ANOVA/ ) [34] . All the DNA microarray data have been deposited to the NCBI Gene Expression Omnibus (GEO, http://www.ncbi.nlm.nih.gov/geo/ ) and are accessible through GEO Series accession number (GSE26278) and the NIA Array Analysis software website ( http://lgsun.grc.nia.nih.gov/ANOVA/ ) [34] . ES cell injection into 2N or tetraploid (4N) blastocysts CD1 females (Charles River, 8–12-week old) were used for superovulation by PMSG (Sigma) followed 48 h later by hCG (Sigma) administration. After hCG administration, females were mated with males of the same strain and 2-cell embryos were collected by flushing oviducts. Recovered embryos were cultured in KSOM (Millipore) medium for 3 days at 37 °C in 5% CO 2 . Collected 2-cell embryos were directly transferred into 0.3 M Mannitol solution and aligned automatically by alternate current pulse in an electrofusion chamber. Then two direct current pulses with 140 V mm −1 were applied for 40 μs using LF101 Electro Cell Fusion Generator. Fused embryos (4N) that have one blastomere were collected at 60 min cultivation and then continued to culture in KSOM medium till they reached the blastocyst stage. A single ES cell or 10–15 ES cells were injected into 2N or 4N blastocysts to assess their developmental potency and then transferred to E2.5 recipient females. To study the effects of Tmx on ES cells, ES cells were cultured in the presence of 200 nM Tmx for 2–3 days before injection. Telomere measurement by quantitative real-time PCR Genomic DNA was extracted from 10 6 cells in biological triplicates and quantified by Nanodrop. Average telomere length ratio was measured from total genomic DNAs using a real-time PCR assay, as previously described [7] , [35] . PCR reactions were performed on the 7500 real-time PCR System (Applied Biosystems) using telomeric primers, control single-copy gene Rplp0 and PCR settings as previously described [35] . Fold induction was calculated by the ΔΔCt method [30] . Immunostaining of Zscan4 ES cells were cultured on the12-well plate, washed by PBS, fixed for 10 min with 4% paraformaldehyde, washed by PBS twice and then treated with 0.25% NP-40 for the permeabilization. Saponin block solution (1% BSA, 10% FBS, 0.2% Saponin in PBS) was applied for the blocking for 30 min and then plates were incubated overnight at 4 °C with rabbit anti-Zscan4 antibodies [7] . Accession codes Microarray data have been deposited in the NCBI Gene Expression Omnibus under accession code GSE26278 . How to cite this article: Amano, T. et al. Zscan4 restores the developmental potency of embryonic stem cells. Nat. Commun. 4:1966 doi: 10.1038/ncomms2966 (2013).